Functional reconstitution of mitochondrial Fe/S cluster synthesis on Isu1 reveals the involvement of ferredoxin Maturation of iron–sulphur (Fe/S) proteins involves complex biosynthetic machinery. In vivo synthesis of [2Fe–2S] clusters on the mitochondrial scaffold protein Isu1 requires the cysteine desulphurase complex Nfs1-Isd11, frataxin, ferredoxin Yah1 and its reductase Arh1. The roles of Yah1–Arh1 have remained enigmatic, because they are not required for in vitro Fe/S cluster assembly. Here, we reconstitute [2Fe–2S] cluster synthesis on Isu1 in a reaction depending on Nfs1-Isd11, frataxin, Yah1, Arh1 and NADPH. Unlike in the bacterial system, frataxin is an essential part of Fe/S cluster biosynthesis and is required simultaneously and stoichiometrically to Yah1. Reduced but not oxidized Yah1 tightly interacts with apo-Isu1 indicating a dynamic interaction between Yah1–apo-Isu1. Nuclear magnetic resonance structural studies identify the Yah1–apo-Isu1 interaction surface and suggest a pathway for electron flow from reduced ferredoxin to Isu1. Together, our study defines the molecular function of the ferredoxin Yah1 and its human orthologue FDX2 in mitochondrial Fe/S cluster synthesis. Proteins with iron–sulphur (Fe/S) co-factors play important roles in fundamental cellular processes such as respiration, amino-acid and cofactor metabolism, DNA metabolism and the regulation of environmental responses [1] , [2] , [3] . In eukaryotic cells, Fe/S clusters are synthesized and inserted into apoproteins by the mitochondrial ISC (iron–sulphur cluster assembly) and the cytosolic cytosolic iron–sulphur protein assembly (CIA) machineries [4] , [5] , [6] , [7] . The ISC machinery is comprised of 17 known proteins most of which have been inherited from their bacterial ancestor [8] , [9] , [10] . Many of the ISC and CIA components are essential for cell viability, underscoring the importance of Fe/S proteins and their biogenesis for the eukaryotic cell. The essentiality of the biosynthesis process is explained by cytosolic and nuclear Fe/S proteins involved in, for example, protein translation, DNA synthesis and repair and other aspects of genome stability and hence has implications for diseases including various forms of cancer [11] , [12] . Mutations in many mitochondrial ISC genes cause neurodegenerative, haematological and metabolic diseases with complex clinical and biochemical phenotypes [6] , [13] , [14] , [15] . Recent studies suggest that both the components and mechanisms of Fe/S protein biogenesis are conserved from yeast to man, making mechanistic studies in the yeast model highly relevant for human biology. The close evolutionary relationship of bacterial and mitochondrial Fe/S protein biogenesis suggests mechanistic similarities of the two pathways, but recent reports also indicate characteristic differences (see below). Mitochondrial (and bacterial) Fe/S protein maturation can be divided into three major steps; the de novo synthesis of a [2Fe–2S] cluster on the scaffold protein Isu1 (bacterial IscU); the release of the cluster from Isu1 by a dedicated Hsp70 chaperone system and its transient binding to Fe/S transfer proteins [16] ; the target-specific insertion of the cluster into apoproteins [4] , [8] , [10] , [17] , [18] . All these steps are assisted by dedicated ISC proteins. The first step crucially requires the cysteine desulphurase complex Nfs1-Isd11 (bacterial IscS; no Isd11 homologue known) that releases sulphur from cysteine by generating a Nfs1-bound persulphide (-SSH) intermediate [19] . Frataxin (yeast Yfh1) is crucial for mitochondrial Fe/S protein biogenesis, and has been proposed to serve as an iron donor and/or positive regulator of the desulphurase enzyme [20] , [21] , [22] . In Salmonella , a frataxin homologue also facilitates Fe/S protein assembly [23] , yet the Escherichia coli frataxin homologue CyaY inhibits Fe/S cluster synthesis in vitro and was suggested to be a negative regulator [24] . In vivo studies have further demonstrated the involvement of the mitochondrial ferredoxin reductase (FDXR) Arh1 and the [2Fe–2S] ferredoxin Yah1 (refs 25 , 26 , 27 , 28 , 29 ). Likewise, an in vivo function in bacterial Fe/S protein biogenesis has been documented for the Yah1 equivalent termed Fdx [30] , [31] . The current work is concentrated on the role of mitochondrial ferredoxin–FDXR as a potential electron transfer chain in Fe/S protein biogenesis. So far, no interaction partner of Yah1 within the mitochondrial ISC system, apart from Arh1, has been described, thus leaving open which ISC protein may accept the electrons. Two steps of this complex biosynthetic process may need the supply of electrons, namely the reduction of the persulphide sulphur (S 0 ) to the sulphide (S 2− ) present in Fe/S clusters and/or the fusion of two [2Fe–2S] to a [4Fe–4S] cluster [8] . In vivo , the latter reaction depends on the late-acting ISC proteins Isa1–Isa2–Iba57 (refs 10 , 32 , 33 ). A role of the ferredoxin chain in the first step is supported by the impaired in vivo Fe/S cluster assembly on Isu1 upon depletion of Yah1 [27] . Consistent with this, bacterial Fdx, both in reduced and oxidized form, was recently shown to interact with IscS [34] . Mixing of reduced Fdx with IscS, IscU, Cys and iron supported the oxidation of Fdx and led to Fe/S cluster formation on IscU. Surprisingly, oxidation of Fdx was already seen upon addition of IscS and Cys only, that is, in the absence of Fe/S cluster formation on IscU precluding mechanistic perceptions on the role of bacterial ferredoxin. Importantly, in vitro Fe/S cluster synthesis on mitochondrial Isu1 does not depend on Yah1, likely due to the presence of the non-physiological reductant dithiothreitol (DTT), which is an essential part of all in vitro Fe/S cluster synthesis assays described so far. Because DTT mediates the reductive release of sulphide from Nfs1–SSH [35] , Fe/S cluster synthesis in previous in vitro reactions may originate from free sulphide rather than Nfs1-bound persulphide. Consequently, DTT-assisted pathways may not fully reflect the physiological situation. To define the putative role of Yah1 in mitochondrial Fe/S cluster synthesis, we develop a DTT-free, yet Yah1-dependent in vitro reconstitution system. Six ISC members efficiently and rapidly assist Fe/S cluster generation in the absence of DTT, as found in the physiological biosynthesis pathway in vivo . Moreover, the primary, high-affinity partner of reduced Yah1 is identified as apo-Isu1 by various methods including microscale thermophoresis (MST) and nuclear magnetic resonance (NMR). Together, our study elucidates a crucial role of Yah1 and its reductase Arh1 in mitochondrial de novo Fe/S cluster synthesis on the scaffold protein Isu1. Fe/S cluster synthesis on Isu1 requires the ferredoxin Yah1 To explore the role of mitochondrial ferredoxin Yah1 in Fe/S cluster assembly, we used time-resolved circular dichroism (CD) spectroscopy for monitoring [2Fe–2S] cluster formation on the scaffold protein Isu1 (ref. 36 ). The Saccharomyces cerevisiae cysteine desulphurase complex Nfs1-Isd11, frataxin Yfh1, ferredoxin Yah1 and the scaffold Isu1 were overproduced and purified from E. coli ( Supplementary Fig. 1 ). Since yeast Isu1 tended to aggregate, we mostly employed its stably folded orthologue CtIsu1 from the thermophilic fungus Chaetomium thermophilum [37] . CtIsu1 could functionally replace its S. cerevisiae counterpart, although complementation was only partial as previously found for E. coli IscU or human IscU [38] ( Supplementary Fig. 2 ). Since functional yeast Arh1 is difficult to obtain [39] , we purified human FDXR, which can transfer its electrons efficiently to both yeast and the two human ferredoxins FDX1 and FDX2 (ref. 28 ) ( Supplementary Fig. 3 ). The Fe/S cluster synthesis reaction was carried out anaerobically in the presence of reduced iron, cysteine and NADPH. Upon mixing of stoichiometric amounts of Nfs1-Isd11, Yfh1, Yah1 and FDXR with the scaffold proteins Isu1 or CtIsu1, a Fe/S cluster formed within seconds. To allow time-resolved experiments, these proteins were mixed at 1:5:5:1:100 molar ratios. The reaction was started by addition of 0.5 mM cysteine, and a [2Fe–2S] cluster formed over minutes as indicated by a characteristic CD spectral peak at 431 nm ( Fig. 1a,b ). The spectral contribution of the [2Fe–2S] protein Yah1 to the overall signal was minimal. The CD spectrum recorded after 30 min was virtually identical to that of holo-CtIsu1 that was chemically reconstituted in the presence of iron and sulphide ions ( Fig. 1b ; Supplementary Fig. 4 ). In the latter case, the CD spectral changes were saturated at 1 equivalent of each iron and sulphide per CtIsu1 monomer, consistent with the formation of a [2Fe–2S] cluster per CtIsu1 dimer. Likely, the [2Fe–2S] cluster is bound in a bridging fashion between two CtIsu1 monomers. 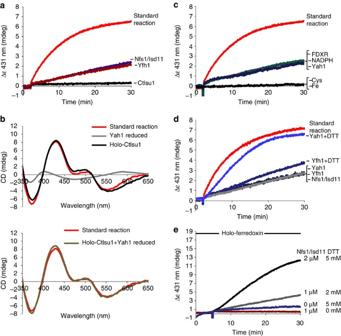Figure 1: Ferredoxin Yah1 supports Nfs1-Isd11-assisted Fe/S cluster synthesis on Isu1. (a–d)De novoFe/S cluster formation onC. thermophilumIsu1 (CtIsu1) was monitored by time-resolved CD spectroscopy under anaerobic conditions at 30 °C. Standard reconstitution mixtures (red lines) contained 100 μM apo-CtIsu1, 1 μM Nfs1-Isd11, 5 μM Yfh1, 5 μM Yah1 and 1.0 μM FDXR in buffer A. In some reconstitution reactions individual components were omitted as indicated. Reactions were started by addition of 0.5 mM cysteine, and the CD signal changes at 431 nm were recorded (a,c,d). In part (b) the full CD spectrum of a standard reaction was recorded after 30 min, and compared with CD spectra of 100 μM chemically reconstituted holo-CtIsu1 (100 μM), reduced Yah1 (5 μM) and the sum of the latter two spectra. (d) The standard reaction was compared with reactions lacking Yah1 or Yfh1, but instead containing 2 mM DTT as indicated (note the initial rate differences of the standard and the −Yah1+DTT reactions). (e)De novoFe/S cluster formation was performed withSynechococcus sp. apo-ferredoxin (50 μM) instead of CtIsu1 under conditions used ina, in the presence of the indicated concentrations of Nfs1-Isd11 and DTT. The dashed line indicates the CD signal for chemically reconstituted holo-ferredoxin. Figure 1: Ferredoxin Yah1 supports Nfs1-Isd11-assisted Fe/S cluster synthesis on Isu1. ( a – d ) De novo Fe/S cluster formation on C. thermophilum Isu1 (CtIsu1) was monitored by time-resolved CD spectroscopy under anaerobic conditions at 30 °C. Standard reconstitution mixtures (red lines) contained 100 μM apo-CtIsu1, 1 μM Nfs1-Isd11, 5 μM Yfh1, 5 μM Yah1 and 1.0 μM FDXR in buffer A. In some reconstitution reactions individual components were omitted as indicated. Reactions were started by addition of 0.5 mM cysteine, and the CD signal changes at 431 nm were recorded ( a , c , d ). In part ( b ) the full CD spectrum of a standard reaction was recorded after 30 min, and compared with CD spectra of 100 μM chemically reconstituted holo-CtIsu1 (100 μM), reduced Yah1 (5 μM) and the sum of the latter two spectra. ( d ) The standard reaction was compared with reactions lacking Yah1 or Yfh1, but instead containing 2 mM DTT as indicated (note the initial rate differences of the standard and the −Yah1+DTT reactions). ( e ) De novo Fe/S cluster formation was performed with Synechococcus sp . apo-ferredoxin (50 μM) instead of CtIsu1 under conditions used in a , in the presence of the indicated concentrations of Nfs1-Isd11 and DTT. The dashed line indicates the CD signal for chemically reconstituted holo-ferredoxin. Full size image The results above strongly suggested that a [2Fe–2S] cluster can be synthesized on the Isu1 scaffold in the absence of DTT. To biochemically dissect the requirements of Fe/S cluster formation, we omitted individual constituents. A >10-fold slower ‘background’ CD signal developed in the absence of the sulphur donor Nfs1-Isd11 or of Yfh1 ( Fig. 1a ). The background reaction was dependent on the addition of CtIsu1, cysteine and iron, and therefore likely represents a non-enzymatic, chemical Fe/S cluster formation on Isu1 (ref. 22 ) ( Fig. 1a,c ). Importantly, in the absence of NADPH, FDXR or Yah1 no CD signal change was observed above the background (that is, the absence of Nfs1-Isd11 or Yfh1) ( Fig. 1c ). This result demonstrates the strict requirement of the Yah1 electron transfer chain for Nfs1-Isd11-catalysed [2Fe–2S] cluster synthesis on Isu1. The participation of these six ISC proteins in Fe/S cluster synthesis in vitro reflects previous physiological findings. Addition of DTT, a reagent causing the reductive release of sulphide from the Nfs1-bound persulphide group [35] , to reaction mixtures lacking Yah1 produced almost the same amount of Fe/S cluster on CtIsu1 (after 30 min) as our standard reaction ( Fig. 1d ). However, the DTT-driven reaction occurred with a significant lag phase in comparison with the Yah1-assisted reaction. Most likely, this delay in Fe/S cluster synthesis reflects the time needed for DTT-mediated production of free sulphide before efficient Fe/S cluster formation can occur. While Yfh1 was essential for Yah1-mediated Fe/S cluster biogenesis in the absence of DTT, slow yet significant Fe/S cluster synthesis was observed in the Yfh1-free, DTT-containing reaction ( Fig. 1d ), a result in keeping with recent observations [21] . We conclude that the DTT-assisted Fe/S cluster synthesis on Isu1 occurs mechanistically different from the ferredoxin Yah1-catalysed reaction, although both reactions eventually produce similar amounts of Isu-bound Fe/S cluster. We asked whether Fe/S cluster formation in our reconstitution system specifically depends on the Isu1 scaffold protein or can also occur on other [2Fe–2S] proteins. No specific CD signal change was generated, when DTT-free reconstitution was attempted with a plant-type bacterial apo-ferredoxin (Fdx) as an acceptor protein instead of Isu1 ( Fig. 1e ; Supplementary Fig. 5 ). In contrast, on addition of DTT, a [2Fe–2S] cluster efficiently formed on Fdx ( Fig. 1e ). This reaction was much slower than Fe/S cluster synthesis on Isu1 at the same concentrations of Nfs1-Isd11 and DTT, yet could be accelerated by increasing the amounts of Nfs1-Isd11 and/or DTT. We further tested whether the Fe/S cluster-carrying ISC protein Nfu1 can assemble Fe/S clusters in our reconstitution system. On the basis of our recent in vivo studies this was not expected, because Fe/S cluster assembly on Nfu1 was dependent on Isu1, Ssq1 and Grx5, that is, Nfu1 apparently acts after Isu1 (ref. 40 ). Since holo-Nfu1 was CD-silent, we separated Nfu1 from low-molecular mass compounds after reconstitution by gel filtration, and estimated the amount of Fe/S cluster formation by the absorption ratio of 420 nm (Fe/S cluster) and 279 nm (protein). Fe/S cluster assembly on Nfu1 was not observed with our standard reconstitution reaction ( cf. Fig. 1a ), yet occurred almost as efficiently as after chemical reconstitution, when DTT was added to the reconstitution system ( Supplementary Fig. 6 ). These results clearly document that Fe/S cluster synthesis in our DTT-free system is specific for the scaffold Isu1, and does not occur on other Fe/S proteins. Taken together, we have reconstituted de novo Fe/S cluster synthesis on the mitochondrial scaffold protein Isu1 in a Nfs1-Isd11-dependent reaction that is fully dependent on the Yah1 electron transfer chain and frataxin. Catalysis by a transient Nfs1-Isd11–Yah1–Yfh1–Isu1 complex We next titrated the amounts of individual ISC components to test the influence on the extent and initial rates of de novo Fe/S cluster synthesis on Isu1. The extent of Fe/S cluster formation linearly increased with the Isu1 concentration ( Fig. 2a ). This result is expected for the reaction 2 Fe+2 Cys+2Isu1→[2Fe–2S]−Isu1-dimer+2 Ala, where a stably bound Fe/S cluster is formed on Isu1 as the final (CD visible) product. In contrast, upon varying the Nfs1-Isd11 concentration the rate of Fe/S cluster formation increased in a linear fashion ( Fig. 2b ). At Nfs1-Isd11 concentrations above 2 μM (corresponding to Nfs1:Isu1 molar ratio of 1:50), the reaction became too fast to be reliably evaluated by our experimental setup. The linear Nfs1-Isd11 concentration dependence of Fe/S cluster synthesis demonstrates that the cysteine desulphurase enzyme was rate limiting, since both Yah1 and Yfh1 were present in excess (5 μM). Different concentration dependencies of the Fe/S cluster synthesis rates were obtained upon varying Yah1 or Yfh1. In these cases, the rates initially increased in a linear, concentration-dependent fashion, yet reached saturation at around 1 μM Yah1 or Yfh1 ( Fig. 2c,d ). Since Nfs1-Isd11 was present at 1 μM, this implies that Fe/S cluster synthesis on Isu1 involves the formation of a stoichiometric, rate-limiting complex of Nfs1-Isd11 with both Yah1 and Yfh1. From the concentration-dependent changes of the rates of Fe/S cluster synthesis, apparent dissociation constants ( K d ) for the interaction of Yah1 and Yfh1 with the remainder synthesis complex can be estimated as 0.3±0.1 μM and 0.1±0.05 μM, respectively. Together, these findings suggest that formation of the Isu1-bound [2Fe–2S] cluster involves the catalytic action of Nfs1-Isd11–Yah1–Yfh1, which likely form a transient biosynthetic complex. 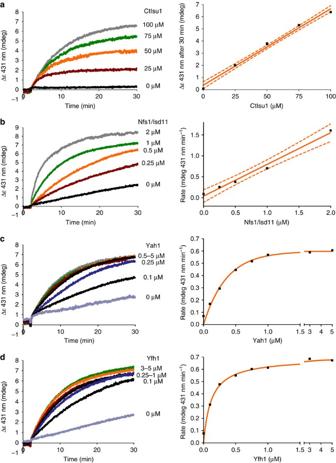Figure 2: Nfs1-Isd11–Yah1–Yfh1 complex is essential for Fe/S cluster formation on Isu1. CD signal changes at 431 nm recording Fe/S cluster formation onC. thermophilumCtIsu1 were monitored in the presence of variable amounts of (a) CtIsu1, (b) Nfs1-Isd11, (c) Yah1 or (d) Yfh1. Panels on the right display the dependence of (a) the extent or (b–d) the initial rates of Fe/S cluster formation on the respective ISC protein concentration. Dashed lines indicate the 95% confidence interval of the linear fits. Error bars indicate the s.e.m. (n≥3). Figure 2: Nfs1-Isd11–Yah1–Yfh1 complex is essential for Fe/S cluster formation on Isu1. CD signal changes at 431 nm recording Fe/S cluster formation on C. thermophilum CtIsu1 were monitored in the presence of variable amounts of ( a ) CtIsu1, ( b ) Nfs1-Isd11, ( c ) Yah1 or ( d ) Yfh1. Panels on the right display the dependence of ( a ) the extent or ( b – d ) the initial rates of Fe/S cluster formation on the respective ISC protein concentration. Dashed lines indicate the 95% confidence interval of the linear fits. Error bars indicate the s.e.m. ( n ≥3). Full size image No free sulphide formed by Yah1-mediated cluster assembly In vivo [2Fe–2S] cluster formation on Isu1 likely occurs via Nfs1- and possibly Isu1-bound persulphide intermediates and not via free sulphide which, however, can be formed in vitro by DTT-mediated reduction of the persulphide present on the cysteine desulphurase Nfs1 (ref. 35 ). To estimate free-sulphide production in our Yah1-dependent, DTT-free assay, we quantified acid-labile sulphide, which includes free sulphide and sulphide present in Fe/S clusters, but not protein-bound persulphide. In our standard reaction ( cf. Fig. 1 ), no significant amounts of acid-labile sulphide were produced above the background determined in the absence of Nfs1-Isd11 ( Fig. 3a ). Part of this background signal originates from the sulphide present in holo-Yah1. In the standard reaction about 0.5 sulphide per added CtIsu1 were generated consistent with a 50% occupancy of an Isu1 dimer with a [2Fe–2S] cluster. Sulphide production was dependent on the presence of Yah1, FDXR, NADPH, Yfh1, Isu1 or iron. This result strongly suggested that Nfs1-Isd11 produced virtually no free sulphide in our DTT-free reconstitution system. Rather, the sulphide developed in our standard reaction is part of the Fe/S cluster generated on Isu1. In contrast, on addition of DTT (with or without Yah1), the acid-labile sulphide content clearly exceeded that found in Yah1-dependent, DTT-free reaction mixtures suggesting that DTT reductively released more sulphide from the Nfs1-bound persulphide intermediate than that found in Isu1-bound Fe/S clusters ( Fig. 3a ). The independence of DTT-mediated sulphide production from Fe/S cluster formation was evident from samples lacking iron. The strong increase in sulphide production compared with iron-containing samples is due to an inhibitory effect of iron on the Nfs1-Isd11 activity. 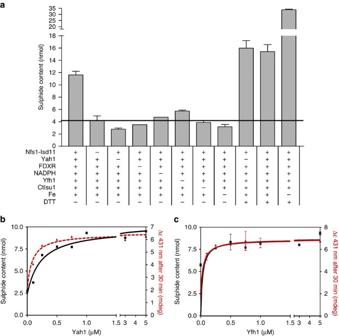Figure 3: No free sulphide is produced during Yah1-mediated Fe/S cluster synthesis. (a) The acid-labile sulphur content was determined in reaction mixtures (200 μl; 20 nmol CtIsu1) under standard conditions containing the indicated components and 2 mM DTT (cf.Fig. 1). (b,c) The acid-labile sulphur content was measured after 30 min for reactions performed with variable amounts of (b) Yah1 or (c) Yfh1 (cf.Fig. 2c,d). For comparison the CD signals at 431 nm at the end of the reactions are shown. Error bars indicate the s.e.m. (n≥3). Figure 3: No free sulphide is produced during Yah1-mediated Fe/S cluster synthesis. ( a ) The acid-labile sulphur content was determined in reaction mixtures (200 μl; 20 nmol CtIsu1) under standard conditions containing the indicated components and 2 mM DTT ( cf. Fig. 1 ). ( b , c ) The acid-labile sulphur content was measured after 30 min for reactions performed with variable amounts of ( b ) Yah1 or ( c ) Yfh1 ( cf. Fig. 2c,d ). For comparison the CD signals at 431 nm at the end of the reactions are shown. Error bars indicate the s.e.m. ( n ≥3). Full size image The conclusion that our DTT-free assay system did not produce any free sulphide and that sulphide production was strictly coupled to Fe/S cluster formation, was further corroborated by varying the Yah1 and Yfh1 concentrations ( cf. Fig. 2c,d ). The extent of acid-labile sulphur formation closely corresponded to the amounts of Isu1-bound Fe/S cluster (as estimated by CD) at all tested Yah1 or Yfh1 concentrations, both signals eventually reaching saturation ( Fig. 3b,c ). This finding strongly suggested that in our Yah1-dependent system acid-labile sulphide is generated only when a Fe/S cluster is formed on Isu1. Taken together, these observations show that sulphide production and ferredoxin-assisted Fe/S cluster synthesis on Isu1 are tightly coupled, and sulphide is not produced in excess, as it is in DTT-mediated reactions. Reduced mitochondrial ferredoxin Yah1 interacts with Isu1 The physiological interaction partner of Yah1 within the mitochondrial ISC assembly machinery has remained elusive. To identify interacting candidate proteins, we first used isolated mitochondria to co-immunoprecipitate proteins associated with a TAP-tagged version of Yah1. Cells with the genomic integration of the C-terminal TAP-tag showed normal growth on yeast extract peptone dextrose medium. Immunostaining of the precipitates for various ISC proteins revealed only Isu1 as a Yah1 interactor ( Fig. 4a ). This in organello interaction was specific, as Isu1 (or any other tested ISC protein) did not co-purify with a TAP-tagged version of Iba57, a late-acting ISC protein [41] . Likewise, Yah1-TAP did not bind to Isd11, that is, the tight complex partner of Nfs1 that could not be analysed directly, because it co-migrated with immunoglobulin G heavy chains on gels. Further evidence for a tight and specific contact of Isu1 and Yah1 was obtained by chemical crosslinking using the zero-length crosslinker EDC ( Fig. 4b ) and gel filtration ( Supplementary Fig. 7 ). 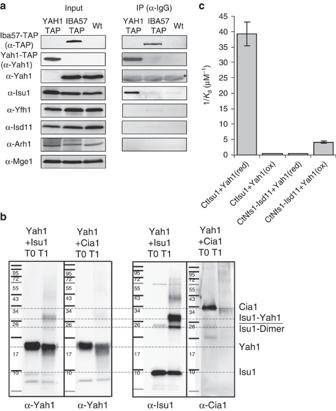Figure 4: The reduced form of Yah1 specifically interacts with Isu1. (a) Isolated mitochondria containing TAP-tagged versions of Yah1 or Iba57 were subjected to affinity purification with immunoglobulin (Ig)G beads. Yah1 and Iba57 were produced at endogenous levels from their own promoters. Mitochondrial lysates (30 μg per lane) and the purified IgG beads were analysed for the presence of the indicated ISC proteins by immunostaining. Wild-type mitochondria (Wt) were included as a specificity control. The asterisk indicates the IgG light chain. (b) Mixtures of purified Yah1 with Isu1 or Cia1 were treated with the zero-length crosslinker EDC. After quenching of the reaction, the proteins were separated by SDS–polyacrylamide gel electrophoresis and analysed by immunostaining for the indicated proteins (α). (c) Yah1 was used as isolated (Yah1(ox)) or reduced with dithionite (Yah1(red)), and mixed at increasing concentrations with 200 nM fluorescently labelled CtIsu1 or CtNfs1-Isd11. Microscale thermophoresis experiments were performed, and dissociation constants (Kd) were determined (Supplementary Fig. 8). Error bars indicate the s.d. (n=6). Figure 4: The reduced form of Yah1 specifically interacts with Isu1. ( a ) Isolated mitochondria containing TAP-tagged versions of Yah1 or Iba57 were subjected to affinity purification with immunoglobulin (Ig)G beads. Yah1 and Iba57 were produced at endogenous levels from their own promoters. Mitochondrial lysates (30 μg per lane) and the purified IgG beads were analysed for the presence of the indicated ISC proteins by immunostaining. Wild-type mitochondria (Wt) were included as a specificity control. The asterisk indicates the IgG light chain. ( b ) Mixtures of purified Yah1 with Isu1 or Cia1 were treated with the zero-length crosslinker EDC. After quenching of the reaction, the proteins were separated by SDS–polyacrylamide gel electrophoresis and analysed by immunostaining for the indicated proteins (α). ( c ) Yah1 was used as isolated (Yah1(ox)) or reduced with dithionite (Yah1(red)), and mixed at increasing concentrations with 200 nM fluorescently labelled CtIsu1 or CtNfs1-Isd11. Microscale thermophoresis experiments were performed, and dissociation constants ( K d ) were determined ( Supplementary Fig. 8 ). Error bars indicate the s.d. ( n =6). Full size image Yah1 is predicted to interact in its reduced state with Isu1 to productively deliver electrons for Fe/S cluster synthesis. The influence of the Yah1 redox state for Isu1 interaction was addressed by MST, an equilibrium method to quantitate protein interactions with binding partners [42] . Increasing amounts of reduced or oxidized Yah1 were mixed with fluorescently labelled CtIsu1 and the thermophoretic behaviour was followed. CtIsu1 strongly interacted with reduced Yah1 ( K d =25 nM), yet 100-fold weaker with oxidized Yah1 ( Fig. 4c ; Supplementary Fig. 8 ). This result demonstrates a preferential interaction of Isu1 with reduced Yah1, thus facilitating electron transfer during de novo Fe/S cluster synthesis. We further used thermophoresis to investigate the potential interaction between Yah1 and Nfs1, since the bacterial counterparts were reported to form a complex [34] . Reduced Yah1 showed only a weak interaction with Nfs1-Isd11, in the K d range of the complex of oxidized Yah1 and Isu1 ( Fig. 4c ). Surprisingly, a 10-fold higher affinity was observed for oxidized Yah1 and Nfs1-Isd11, suggesting a dynamic rearrangement of Yah1 within the ISC biosynthetic complex after electron transfer. Notably, the binding between reduced Yah1 and apo-Isu1 was still 10-fold stronger than that between oxidized Yah1 and Nfs1-Isd11, emphasizing the physiological relevance of reduced Yah1–apo-Isu1 interaction for initiating Fe/S cluster synthesis. Structural characterization of Yah1 interaction with Isu1 To gain atomic insight into the interaction between reduced Yah1 and Isu1, we performed a NMR characterization of S. cerevisiae Yah1 (residues 58–172), determining the NMR resonance assignment and the solution structures of its reduced and oxidized forms. 1 H– 15 N heteronuclear single-quantum coherence (HSQC) spectra for both Yah1 redox states showed well-dispersed amide resonances, indicating a well-folded protein. Similar signal patterns of both states excluded a major overall conformational alteration during the redox reaction. Relaxation analysis of oxidized Yah1 showed heteronuclear R 1 and R 2 values typical of a monomeric protein of about 13 kDa and positive 15 N( 1 H) nuclear overhauser effect (NOE) values ( Supplementary Fig. 9 ). These results were consistent with a folded, essentially rigid protein. From R 2 / R 1 ratios a correlation time of 6.5±1.2 ns was estimated. This value compares well with the one calculated by HYDRONMR (7.2 ns), and is consistent with the monomeric state of the protein. In both redox states the [2Fe–2S] cluster, bound to Cys 98,104, 107 and 144, produced paramagnetic effects on the NMR spectra, because the magnetic coupling between the iron ions gives rise to ground and/or excited paramagnetic electronic spin states [43] ( Supplementary Fig. 9 ). The fast relaxation of nuclei close to the Fe/S cluster makes their detection impossible with standard approaches. To overcome this problem, NMR experiments tailored to detect fast relaxing signals were performed, which rely on 13 C direct detection and fast cycling [44] . This allowed recording of high numbers of scans with concomitant saturation of the slow relaxing signals. Thereby, backbone resonance assignment for 92 and 88 out of 115 amino-acid residues was obtained for oxidized and reduced Yah1, respectively. The undetected residues (stretches 96–108 and 143–145 in oxidized Yah1; 95–109 and 142–146 in reduced Yah1) were all located close to the [2Fe–2S] cluster. The NH signals in the C-terminal region (160–169), that is, far from the cluster, were also extensively broadened suggesting an unstructured polypeptide chain. In contrast, the last three residues (170–172) again showed NH signals and were characterized by low values for heteronuclear NOEs, typical for a random coil conformation ( Supplementary Fig. 9 ). The assignment of the unstructured region for both redox states was achieved by 13 C direct detection NMR experiments that confirmed the random coil conformation. The overall structure of Yah1 showed a compact (α+β) fold in both redox states, yet in addition to the four α-helices and four β-strands typical for crystal structures of [2Fe–2S] ferredoxins such as human FDX2, our solution structure encompassed the C-terminal region ( Fig. 5a ; Supplementary Fig. 10 ; Supplementary Tables 1 and 2 ). 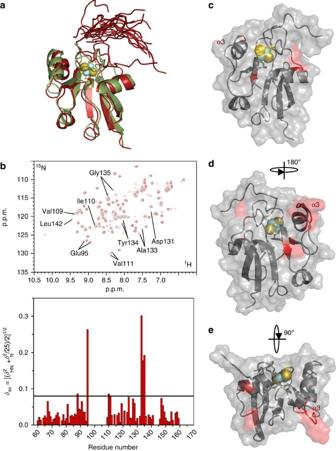Figure 5: Ferredoxin Yah1 shows structural changes upon interaction with Isu1. (a) Superposition of the crystal structure of the human FDX2 in green (pdb accession code: 2Y5C) with the NMR solution structure of yeast Yah1 in red (pdb: 2MJE (reduced) and 2MJD (oxidized)). The [2Fe–2S] clusters of both redox states are depicted in yellow (sulphur) and silver (iron), with the coordinating cysteine residues represented by sticks. Yah1 shows a common ferredoxin fold with an ultra-flexible C terminus and a rigid core. (b) Superposition of the HSQC spectra of reduced Yah1 alone (grey) and in complex with CtIsu1 (red). At least six Yah1 residues show a chemical shift upon interaction with CtIsu1. This is evident from the weighted-average chemical shift differences ΔHN(that is, ([(δH)2+(δN/5)2]/2)1/2, whereδHandδNare chemical shift differences for1H and15N, respectively) of reduced Yah1 without and with bound apo-CtIsu1 (bottom). The horizontal black line indicates the average chemical shift variation plus one s.d. upon Isu1 addition. (c–e) The surface of the Yah1 solution structure in three different orientations is presented by mesh. All Yah1 residues (red), which show a chemical shift upon interaction with CtIsu1, are located close to each other near helix α3. Figure 5: Ferredoxin Yah1 shows structural changes upon interaction with Isu1. ( a ) Superposition of the crystal structure of the human FDX2 in green (pdb accession code: 2Y5C) with the NMR solution structure of yeast Yah1 in red (pdb: 2MJE (reduced) and 2MJD (oxidized)). The [2Fe–2S] clusters of both redox states are depicted in yellow (sulphur) and silver (iron), with the coordinating cysteine residues represented by sticks. Yah1 shows a common ferredoxin fold with an ultra-flexible C terminus and a rigid core. ( b ) Superposition of the HSQC spectra of reduced Yah1 alone (grey) and in complex with CtIsu1 (red). At least six Yah1 residues show a chemical shift upon interaction with CtIsu1. This is evident from the weighted-average chemical shift differences Δ HN (that is, ([( δ H ) 2 +( δ N /5) 2 ]/2) 1/2 , where δ H and δ N are chemical shift differences for 1 H and 15 N, respectively) of reduced Yah1 without and with bound apo-CtIsu1 (bottom). The horizontal black line indicates the average chemical shift variation plus one s.d. upon Isu1 addition. ( c – e ) The surface of the Yah1 solution structure in three different orientations is presented by mesh. All Yah1 residues (red), which show a chemical shift upon interaction with CtIsu1, are located close to each other near helix α3. Full size image To explore the regions of interaction between reduced Yah1 and CtIsu1, we performed NMR titrations through 1 H– 15 N HSQC spectra under anaerobic conditions. In the presence of CtIsu1, spectral changes were observed only for reduced but not for oxidized Yah1, consistent with the affinity measurements by thermophoresis ( cf. Fig. 4c ). Residues of Yah1 with largest variation were Ala133, Tyr134, Gly135, Gln88, Glu95 and Ile110 ( Fig. 5b ). These residues are located in a region surrounding the [2Fe–2S] cluster on the helix α3 side of the protein ( Fig. 5c–e ), and may represent the Yah1–CtIsu1 interaction region. Conspicuously, a group of acidic residues (Gln88, Glu95, Asp128 and Asp131) in the helix α3 is present in the interaction region, suggesting a key role of these electrostatic residues in electron transfer to Isu1. Only human FDX2 assists Fe/S cluster assembly on Isu1 Human cells possess two distinct mitochondrial ferredoxins, the adrenodoxin FDX1, which functions in steroid hormone production and is mainly expressed in adrenal gland and kidney cells, and the ubiquitously expressed FDX2 (ref. 28 ). To analyse their functional specificity, we replaced Yah1 in our standard reaction ( cf. Fig. 1 ) by purified human FDX1 or FDX2. FDX1 is highly efficient in cortisol production [28] , yet was unable to support de novo Fe/S cluster synthesis on Isu1 above the background ( Fig. 6a ). In contrast, FDX2 could replace yeast Yah1 at virtually identical efficiency. This result shows a specific role of human FDX2, but not of FDX1, in cellular Fe/S protein maturation. 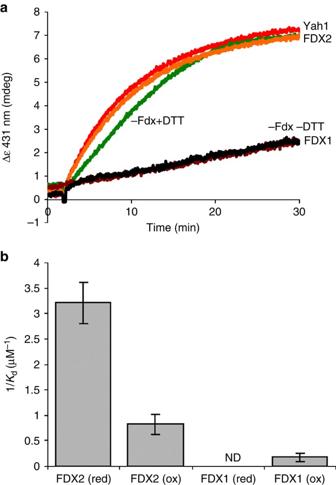Figure 6: Human FDX2, but not FDX1, mediates Fe/S cluster synthesis on Isu1. (a)De novoFe/S cluster formation on CtIsu1 was monitored by time-resolved CD spectroscopy under standard conditions as inFig. 1in the presence of eitherS. cerevisiaeYah1, human FDX1 or human FDX2 as indicated. Control reactions were performed in the absence of any ferredoxin (−Fdx) with or without DTT. (b) Human FDX1 and FDX2 were reduced with dithionite (red) or used as isolated (ox), and mixed with 200 nM fluorescently labelled CtIsu1 (cf.Fig. 4c). Microscale thermophoresis experiments were performed, and dissociation constants (Kd) were determined (Supplementary Fig. 11). Error bars indicate the s.d. (n≥3). ND, not determinable. Figure 6: Human FDX2, but not FDX1, mediates Fe/S cluster synthesis on Isu1. ( a ) De novo Fe/S cluster formation on CtIsu1 was monitored by time-resolved CD spectroscopy under standard conditions as in Fig. 1 in the presence of either S. cerevisiae Yah1, human FDX1 or human FDX2 as indicated. Control reactions were performed in the absence of any ferredoxin (−Fdx) with or without DTT. ( b ) Human FDX1 and FDX2 were reduced with dithionite (red) or used as isolated (ox), and mixed with 200 nM fluorescently labelled CtIsu1 ( cf. Fig. 4c ). Microscale thermophoresis experiments were performed, and dissociation constants ( K d ) were determined ( Supplementary Fig. 11 ). Error bars indicate the s.d. ( n ≥3). ND, not determinable. Full size image Finally, equilibrium titrations with MST showed that reduced FDX2 bound fourfold stronger to CtIsu1 than oxidized FDX2 ( Fig. 6b ; Supplementary Fig. 11a ). The binding constant was 10-fold weaker than that of the reduced Yah1–CtIsu1 complex, possibly reflecting the evolutionary distance of this protein pair. In contrast, FDX1 showed hardly any binding to CtIsu1, in neither the reduced nor oxidized form ( Fig. 6b ; Supplementary Fig. 11b ). We conclude that human FDX2 is part of the electron transport chain required for de novo mitochondrial Fe/S protein biogenesis, while FDX1 function is dedicated to steroid metabolism in the adrenal gland. Here, we have reconstituted the de novo synthesis of a [2Fe–2S] cluster on the scaffold protein Isu1, the crucial initial step of mitochondrial Fe/S protein biogenesis. In vivo studies have provided evidence for a dependence of this reaction on the cysteine desuphurase complex Nfs1-Isd11, frataxin Yfh1 and the ferredoxin Yah1 (refs 27 , 45 ). However, previous in vitro reconstitution experiments of mitochondrial Fe/S cluster synthesis have failed to reveal the requirement of the ferredoxin electron transfer chain, since reaction mixtures contained the artificial reductant DTT (see, for example, refs 46 , 47 ). Hence, it was not possible to address the crucial requirement for reducing equivalents in Fe/S cluster synthesis, thus precluding mechanistic perceptions of the role of mitochondrial ferredoxin. Our time-resolved in vitro reconstitution system for Fe/S cluster synthesis on mitochondrial Isu1 crucially requires the electron transfer chain NADPH–FDXR–ferredoxin, yet is independent of DTT. When carried out with stoichiometric amounts of Nfs1-Isd11, Yfh1, Yah1, FDXR and Isu1 above 10-micromolar concentrations, the reaction completed within seconds at high yield. The requirement of all ISC components identified in vivo for mitochondrial Fe/S cluster synthesis on Isu1, the rapid reconstitution rate and the high efficiency strongly suggest that our experimental approach occurs similarly to the physiological pathway. To gain mechanistic insights into the synthesis reaction, the majority of our experiments were performed at lower (that is, catalytic) concentrations of Nfs1-Isd11, which proved to be the rate-limiting enzyme for Fe/S cluster synthesis on Isu1. Both frataxin and ferredoxin Yah1 were needed in stoichiometric amounts relative to Nfs1-Isd11, suggesting that the complex of Nfs1-Isd11–Yfh1–Yah1 determines the overall rate of Fe/S cluster synthesis on Isu1. This finding suggests that both Yfh1 and Yah1 need to be present simultaneously at Nfs1-Isd11–Isu1, since an alternating binding of Yfh1 and Yah1 during the catalytic cycle would not require stoichiometric amounts.This indicates that the catalytic entity for Fe/S cluster synthesis on Isu1 is the complex of Nfs1-Isd11–Yfh1–Yah1. Clearly, this dynamic complex may interact only transiently with Isu1, which was present in large (>20-fold) excess and thus has to dissociate from the other proteins after holo-formation. The requirement of a five-membered biosynthetic entity clearly distinguishes the mitochondrial Fe/S cluster synthesis system from the bacterial one, where Fdx and CyaY (frataxin) were suggested to occupy overlapping binding sites on IscS and thus mutually bind to the desulphurase [34] , [48] . On the basis of these fundamental differences, bacterial and mitochondrial Fe/S cluster synthesis surprisingly differ at the molecular level. Further characteristics discriminate mitochondrial and bacterial ISC assembly pathways, despite the striking evolutionary relationship. Bacterial CyaY inhibits rather than stimulates Fe/S cluster synthesis in vitro [24] , and hence was suggested to act as a negative regulator. The inhibitory effect depended on the source of the desulphurase, because bacterial IscS was also inhibited by (high amounts of) human frataxin. In contrast, the Salmonella CyaY homologue was required in vivo for normal Fe–S cluster metabolism [23] . Notably, the in vitro studies on bacterial CyaY were performed in the presence of DTT, which may affect the reaction mechanism (see below and ref. 22 [22] ). It is evident from these criteria that some aspects of mitochondrial and bacterial de novo Fe/S cluster synthesis may be mechanistically different. The independence of previous in vitro assays on the ferredoxin electron transfer chain can be attributed to the presence of the reductant DTT. In our reconstitution system, DTT could efficiently replace the electron transfer chain NADPH, FDXR and Yah1. Although the yields of Fe/S cluster formation on Isu1 in the presence of DTT or in the Yah1-dependent system were virtually identical, the initial rates of both reactions differed characteristically. While the ferredoxin-dependent reaction initiated immediately after adding cysteine, the DTT-driven synthesis started off only after a short lag phase. These different time courses indicate that Fe/S cluster formation on Isu1 occurs along mechanistically different pathways in the two assay systems. How can this be explained? In all likelihood, DTT reduces the Nfs1-bound persulphide to free sulphide, which is subsequently used for chemical Fe/S cluster synthesis. While the DTT- and Nfs1-dependent in vitro sulphide generation is well documented [35] , physiological Fe/S cluster formation is believed to occur via persulphide transfer from Nfs1 to Isu1 (ref. 8 ), followed by reduction of the Isu1 persulphide to an Fe/S cluster-integrated sulphide by direct protein interaction with Yah1. Consistent with such a persulphide relay scenario [17] , [49] , we did not observe the production of free sulphide in the Yah1-dependent reaction. All detectable acid-labile sulphide was derived from the Fe/S clusters synthesized on Isu1. The ISC protein dependencies and time courses of Fe/S cluster synthesis and of acid-labile sulphide production were virtually identical, consistent with a tight coupling of both reactions. Overall, these results suggest that Fe/S cluster synthesis in the presence of DTT may not fully reflect the in vivo situation, and rather may occur like a chemical reconstitution with inorganic iron and sulphide ions. This explains well why a bacterial non-scaffold Fe/S protein could not be matured via the Yah1-dependent, DTT-free pathway, but only in the presence of DTT ( Fig. 1e ). A similar observation was made for the non-scaffold mitochondrial ISC protein Nfu1 ( Supplementary Fig. 6 ). Collectively, all these criteria show that the Yah1-dependent Fe/S cluster synthesis on Isu1 may occur similar to the physiological pathway. We have obtained several lines of in vivo and in vitro evidence to suggest that Yah1 dynamically and tightly interacts with Isu1. In organello co-immunoprecipitation identified a complex of these two ISC components, yet no stable interaction was observed between Yah1 and other ISC components, such as Nfs1-Isd11 and Yfh1. In vitro , the specific interaction between Yah1 and Isu1 was documented by chemical crosslinking, gel filtration, MST-binding studies and NMR structural analyses. In particular, the novel method of MST allowed equilibrium titrations with reduced or oxidized Yah1. This method identified a strong affinity ( K d =25 nM) between reduced Yah1 and apo-Isu1. A 100-fold weaker affinity was observed for oxidized Yah1 and apo-Isu1 strongly suggesting that upon electron delivery by Yah1 its interaction with Isu1 is loosened. The high preference of apo-Isu1 for reduced Yah1 provides strong evidence for the in vivo relevance of the encounter of the two proteins. Our reconstitution system forms the basis for the future elucidation of the biochemical mechanism of the reduction step by biophysical methods. On the basis of our findings an obvious candidate for reduction is the (putative) persulphide intermediate of Isu1, which seems to be short-lived and may require special technology for detection. However, the close vicinity of the Nfs1-bound persulphide group to Isu1 (as evident from bacterial ISC structures [50] , [51] , [52] ) does not exclude that the ferredoxin-derived electrons are used for reduction of this moiety or another reaction intermediate. Interestingly, Yah1 also interacted with Nfs1-Isd11 in vitro . The thermophoresis data show a higher affinity for oxidized Yah1 with Nfs1-Isd11 compared with Isu1, suggesting that oxidation of Yah1 loosens the interaction with Isu1 and tightens binding with Nfs1-Isd11. These results may suggest a dynamic rearrangement of the five-membered ISC complex during Fe/S cluster formation, where the ferredoxin interacts with both the scaffold and the desulphurase. In fact, the bacterial ferredoxin Fdx was shown to specifically interact with IscS, but this was independent of its redox state [34] , [48] . Furthermore, docking calculations suggest that bacterial Fdx may bind in a cleft between IscS and IscU, which is consistent with our MST interaction studies [48] , [51] . However, since bacterial frataxin (CyaY) is predicted to also bind here at an overlapping site, the mitochondrial and bacterial systems may be distinct at the molecular level (see above). Our NMR structural analyses further extended the insights into the redox state-dependent complex formation between Yah1 and Isu1. A few NMR resonances of reduced but not of oxidized Yah1 were altered by the binding of apo-Isu1, indicating a high specificity of this encounter. In contrast, multiple alterations were observed upon interaction of bacterial Fdx with IscS, which also included non-overlapping regions in the two studies [34] , [48] . Conspicuously, four of the mobile Fdx residues (corresponding to Yah1 I110, A133, Y134 and G135) were also chemically shifted upon Yah1–Isu1 interaction. In contrast to our findings, there were no differences for the two redox states of bacterial Fdx leaving open how Fdx would dissociate from IscS after electron transfer. The chemical shift changes on reduced Yah1 upon incubation with apo-Isu1 may indicate the interaction surface of the two proteins. Contacting residues are essentially hydrophilic, and one of them, Tyr134, could play a key role in the protein–protein interaction. Indeed, in the oxidized structure, it is positioned close to the fully conserved His108 and could form a hydrogen bond with it. This hydrogen bond could be abolished upon reduction, thus inducing the structural changes in this region. These changes could be transferred to the nearby and interacting helix α3 (ref. 53 ). The definition of the interaction region provides a first clue for how the electrons may move from Yah1 towards Isu1, because the hydrophilic interaction surface is close to the embedded [2Fe–2S] cluster of Yah1 ( Fig. 5 ). It will be interesting to resolve the structural arrangement of Isu1 and its Cys ligands to get a complete view of the electron flow. Our biochemical system was also useful to clarify the function of the two human ferredoxins FDX1 (aka adrenodoxin) and FDX2. Deficiency of the latter protein is associated with a mitochondrial muscle myopathy, which is similar to the disorder described for IscU deficiency [6] , [14] , [54] . The similar disease phenotype reassures that both proteins act in the same biochemical step. Sheftel et al. [28] found no evidence for an involvement of FDX1 in Fe/S protein biogenesis, yet could support its well-established, specific role in steroid hormone production. Purified FDX1, but not FDX2, was functional in cytochrome P 450 -mediated generation of cortisol. An additional role of FDX1 in Fe/S protein biogenesis seemed unlikely, because its depletion in HeLa cells did not elicit any defects in cellular Fe/S protein biogenesis, and its overproduction did not restore the severe Fe/S protein defects upon depletion of FDX2 (ref. 28 ). In contrast, RNA interference-mediated depletion of either FDX1 or FDX2 was reported to impair Fe/S protein maturation [29] . In our in vitro system, only FDX2, but not FDX1, could replace yeast Yah1. Both the rates and the efficiency of Fe/S cluster synthesis on Isu1 were similar for Yah1 and FDX2. The results fit nicely to the almost exclusive expression of FDX1 in adrenal gland, while FDX2 is ubiquitously found in virtually all tissues, consistent with its essential function in all cell types [28] . In summary, the two human ferredoxins perform non-exchangeable roles in different biochemical processes in distinct cell types. While the function of Yah1 and FDX2 in Fe/S cluster synthesis on Isu1 is supported by in vivo and in vitro evidence, future studies will have to address the precise electrochemical mechanism of electron transfer. In vitro reconstitution of Fe/S cluster synthesis on Isu1 The samples for in vitro Fe/S cluster synthesis were prepared in a COY anaerobic chamber using freshly dissolved stock solutions. Protein solutions were incubated under anaerobic conditions for at least 1 h before the experiments. The 300-μl standard reaction contained 1 μM Nfs1-Isd11, 5 μM Yfh1, 5 μM Yah1, 1 μM human FDXR and 100 μM of either Isu1 or CtIsu1 in buffer A (25 mM Tris-HCl, pH 8.0, 150 mM NaCl, 2 mM MgCl 2 , 10 μM PLP, 1 mM NADPH, 1 mM sodium ascorbate and 0.3 mM FeCl 2 ). The reaction was transferred to a CD cuvette, sealed tightly and placed at 30 °C in a CD spectrophotometer (J-815, Jasco). After 2 min, the Fe/S cluster synthesis reaction was initiated by the anaerobic addition of 0.5 mM cysteine via a syringe. The CD signal change at 431 nm or full spectra were recorded. Kinetic evaluations of the data were carried out using GraphPad Prism software. Affinity measurements using MST MST was performed on a Monolith NT.115 (NanoTemper Technologies GmbH, Munich, Germany) at 32 or 28 °C (red LED power was set between 60 and 100% and infrared laser power to 80%) [42] . CtIsu1 or CtNfs1-Isd11 (20 μM each) were labelled with the dye NT 647 according to the supplier (NanoTemper Technologies). Two hundred nM CtIsu1 or CtNfs1-Isd11 were titrated with unlabelled Yah1 in 35 mM KP i pH 7.4, 150 mM NaCl. At least six independent MST experiments were recorded at 680 nm and processed by NanoTemper Analysis 1.2.009 and Origin8. Structure determination and interaction analysis by NMR NMR experiments used for resonance assignment and structure calculations for either oxidized or reduced Yah1 were recorded under anaerobic conditions on Bruker AVANCE 500 or BRUKER AVANCE III 950 spectrometers, equipped with cryoprobes, on 0.5 mM 13 C, 15 N-labelled or 15 N-labelled Yah1 samples in 30 mM phosphate buffer, pH 7.0, containing 10% (v/v) D 2 O and 100 mM NaCl. NMR spectra were collected at 298 K, and processed using the standard BRUKER software (Topspin). The structures of both redox states were calculated using the standard NOE-based restraints for the protein part not affected by paramagnetism, while for the paramagnetic region, 13 C paramagnetic longitudinal relaxation rates were measured on both redox states and then translated into cluster– 13 C upper limit distance constraints and used in the structural calculations. 15 N-labelled Yah1 (0.5 mM), either in the oxidized or reduced state, was titrated with increasing amounts of the unlabelled CtIsu1 (0.125–1 mM), and the chemical shift changes were followed in the 1 H– 15 N HSQC NMR spectra, and the differences in chemical shifts of oxidized and reduced Yah1 were accounted for. For further details see Supplementary Methods . Accession codes: Structural coordinates for reduced and oxidized Yah1 have been deposited in the RCSB Protein Data Bank under accession codes 2MJE and 2MJD , respectively. How to cite this article: Webert, H. et al. Functional reconstitution of mitochondrial Fe/S cluster synthesis on Isu1 reveals the involvement of ferredoxin. Nat. Commun. 5:5013 doi: 10.1038/ncomms6013 (2014).